Multi-ancestry study of blood lipid levels identifies four loci interacting with physical activity Many genetic loci affect circulating lipid levels, but it remains unknown whether lifestyle factors, such as physical activity, modify these genetic effects. To identify lipid loci interacting with physical activity, we performed genome-wide analyses of circulating HDL cholesterol, LDL cholesterol, and triglyceride levels in up to 120,979 individuals of European, African, Asian, Hispanic, and Brazilian ancestry, with follow-up of suggestive associations in an additional 131,012 individuals. We find four loci, in/near CLASP1 , LHX1 , SNTA1 , and CNTNAP2 , that are associated with circulating lipid levels through interaction with physical activity; higher levels of physical activity enhance the HDL cholesterol-increasing effects of the CLASP1 , LHX1 , and SNTA1 loci and attenuate the LDL cholesterol-increasing effect of the CNTNAP2 locus. The CLASP1 , LHX1 , and SNTA1 regions harbor genes linked to muscle function and lipid metabolism. Our results elucidate the role of physical activity interactions in the genetic contribution to blood lipid levels. Circulating levels of blood lipids are strongly linked to the risk of atherosclerotic cardiovascular disease. Regular physical activity (PA) improves blood lipid profile by increasing the levels of high-density lipoprotein cholesterol (HDL-C) and decreasing the levels of low-density lipoprotein cholesterol (LDL-C) and triglycerides (TG) [1] . However, there is individual variation in the response of blood lipids to PA, and twin studies suggest that some of this variation may be due to genetic differences [2] . The genes responsible for this variability remain unknown. More than 500 genetic loci have been found to be associated with blood levels of HDL-C, LDL-C, or TG in published genome-wide association studies (GWAS) [3] , [4] , [5] , [6] , [7] , [8] , [9] , [10] , [11] , [12] . At present, it is not known whether any of these main effect associations are modified by PA. Understanding whether the impact of lipid loci can be modified by PA is important because it may give additional insight into biological mechanisms and identify subpopulations in whom PA is particularly beneficial. Here, we report results from a genome-wide meta-analysis of gene–PA interactions on blood lipid levels in up to 120,979 adults of European, African, Asian, Hispanic, or Brazilian ancestry, with follow-up of suggestive associations in an additional 131,012 individuals. We show that four loci, in/near CLASP1 , LHX1 , SNTA1 , and CNTNAP2 , are associated with circulating lipid levels through interaction with PA. None of these four loci have been identified in published main effect GWAS of lipid levels. The CLASP1 , LHX1 , and SNTA1 regions harbor genes linked to muscle function and lipid metabolism. Our results elucidate the role of PA interactions in the genetic contribution to blood lipid levels. Genome-wide interaction analyses in up to 250,564 individuals We assessed effects of gene–PA interactions on serum HDL-C, LDL-C, and TG levels in 86 cohorts participating in the Cohorts for Heart and Aging Research in Genomic Epidemiology (CHARGE) Gene-Lifestyle Interactions Working Group [13] . PA was harmonized across participating studies by categorizing it into a dichotomous variable. The participants were defined as inactive if their reported weekly energy expenditure in moderate-to-vigorous intensity leisure-time or commuting PA was less than 225 metabolic equivalent (MET) minutes per week (corresponding to approximately 1 h of moderate-intensity PA), while all other participants were defined as physically active (Supplementary Data 1 ). The analyses were performed in two stages. Stage 1 consisted of genome-wide meta-analyses of linear regression results from 42 cohorts, including 120,979 individuals of European [ n = 84,902], African [ n = 20,487], Asian [ n = 6403], Hispanic [ n = 4749], or Brazilian [ n = 4438] ancestry (Supplementary Tables 1 and 2 ; Supplementary Data 2 ; Supplementary Note 1 ). All variants that reached two-sided P < 1 × 10 −6 in the Stage 1 multi-ancestry meta-analyses or ancestry-specific meta-analyses were taken forward to linear regression analyses in Stage 2, which included 44 cohorts and 131,012 individuals of European [ n = 107,617], African [ n = 5384], Asian [ n = 6590], or Hispanic [ n = 11,421] ancestry (Supplementary Tables 3 and 4 ; Supplementary Data 3 ; Supplementary Note 2 ). The summary statistics from Stage 1 and Stage 2 were subsequently meta-analyzed to identify lipid loci whose effects are modified by PA. We identified lipid loci interacting with PA by three different approaches applied to the meta-analysis of Stage 1 and Stage 2: (i) we screened for genome-wide significant SNP × PA-interaction effects ( P INT < 5 × 10 −8 ); (ii) we screened for genome-wide significant 2 degree of freedom (2df) joint test of SNP main effect and SNP × PA interaction [14] ( P JOINT < 5 × 10 −8 ); and (iii) we screened all previously known lipid loci [3] , [4] , [5] , [6] , [7] , [8] , [9] , [10] , [11] , [12] for significant SNP × PA-interaction effects, Bonferroni-correcting for the number of independent variants tested ( r 2 < 0.1 within 1 Mb distance; P INT = 0.05/501 = 1.0 × 10 −4 ). 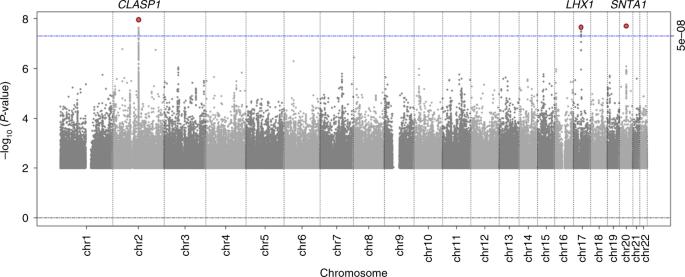Fig. 1 Genome-wide results for interaction with physical activity on HDL cholesterol levels. ThePvalues are two-sided and were obtained by a meta-analysis of linear regression model results (nup to 250,564). Three loci, in/nearCLASP1,LHX1, andSNTA1, reached genome-wide significance (P< 5 × 10−8) as indicated in the plot PA modifies the effect of four loci on lipid levels Three novel loci (>1 Mb distance and r 2 < 0.1 with any previously identified lipid locus) were identified: in CLASP1 (rs2862183, P INT = 8 × 10 −9 ), near LHX1 (rs295849, P INT = 3 × 10 −8 ), and in SNTA1 (rs141588480, P INT = 2 × 10 −8 ), which showed a genome-wide significant SNP × PA interaction on HDL-C in all ancestries combined (Table 1 , Figs. 1 – 4 ). 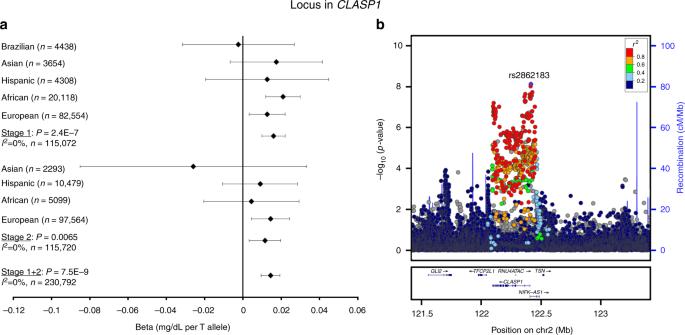Fig. 2 Interaction of rs2862183 inCLASP1with physical activity on HDL cholesterol levels. The beta and 95% confidence intervals in the forest plot (a) is shown for the rs2862183 × physical activity interaction term, i.e., it indicates the increase in logarithmically transformed HDL cholesterol levels in the active group as compared to the inactive group per each T allele of rs2862183. The −log10(Pvalue) in the association plot (b) is also shown for the rs2862183 × physical activity interaction term. ThePvalues are two-sided and were obtained by a meta-analysis of linear regression model results. The figure was generated using LocusZoom (http://locuszoom.org) Higher levels of PA enhanced the HDL cholesterol-increasing effects of the CLASP1 , LHX1 , and SNTA1 loci. A novel locus in CNTNAP2 (rs190748049) was genome-wide significant in the joint test of SNP main effect and SNP × PA interaction ( P JOINT = 4 × 10 −8 ) and showed moderate evidence of SNP × PA interaction ( P INT = 2 × 10 −6 ) in the meta-analysis of LDL-C in all ancestries combined (Table 1 , Fig. 5 ). The LDL-C-increasing effect of the CNTNAP2 locus was attenuated in the physically active group as compared to the inactive group. None of these four loci have been identified in previous main effect GWAS of lipid levels. Table 1 Lipid loci identified through interaction with physical activity ( P INT < 5 × 10 −8 ) or through joint test for SNP main effect and SNP × physical activity interaction ( P JOINT < 5 × 10 −8 ) Full size table Fig. 1 Genome-wide results for interaction with physical activity on HDL cholesterol levels. The P values are two-sided and were obtained by a meta-analysis of linear regression model results ( n up to 250,564). Three loci, in/near CLASP1 , LHX1 , and SNTA1 , reached genome-wide significance ( P < 5 × 10 −8 ) as indicated in the plot Full size image Fig. 2 Interaction of rs2862183 in CLASP1 with physical activity on HDL cholesterol levels. The beta and 95% confidence intervals in the forest plot ( a ) is shown for the rs2862183 × physical activity interaction term, i.e., it indicates the increase in logarithmically transformed HDL cholesterol levels in the active group as compared to the inactive group per each T allele of rs2862183. The −log 10 ( P value) in the association plot ( b ) is also shown for the rs2862183 × physical activity interaction term. The P values are two-sided and were obtained by a meta-analysis of linear regression model results. The figure was generated using LocusZoom ( http://locuszoom.org ) Full size image Fig. 3 Interaction of rs295849 near LHX1 with physical activity on HDL cholesterol levels. The beta and 95% confidence intervals in the forest plot ( a ) is shown for the rs295849 × physical activity interaction term, i.e., it indicates the increase in logarithmically transformed HDL cholesterol levels in the active group as compared to the inactive group per each G allele of rs295849. The −log 10 ( P value) in the association plot ( b ) is also shown for the rs295849 × physical activity interaction term. The P values are two-sided and were obtained by a meta-analysis of linear regression model results. The figure was generated using LocusZoom ( http://locuszoom.org ) Full size image Fig. 4 Interaction of rs141588480 in SNTA1 with physical activity on HDL cholesterol levels. The beta and 95% confidence intervals in the forest plot ( a ) is shown for the rs141588480 × physical activity interaction term, i.e., it indicates the increase in logarithmically transformed HDL cholesterol levels in the active group as compared to the inactive group per each insertion of rs141588480. The –log 10 ( p value) in the association plot ( b ) is also shown for the rs141588480 × physical activity interaction term. While the rs141588480 variant was identified in African-ancestry individuals in Stage 1, the variant did not pass QC filters in the Stage 2 African-ancestry cohorts, due to insufficient sample sizes of these cohorts. The P values are two-sided and were obtained by a meta-analysis of linear regression model results. The figure was generated using LocusZoom ( http://locuszoom.org ) Full size image Fig. 5 Interaction of rs190748049 variant in CNTNAP2 with physical activity on LDL cholesterol levels. The rs190748049 variant was genome-wide significant in the joint test for SNP main effect and SNP × physical activity interaction and reached P = 2 × 10 −6 for the SNP × physical activity interaction term alone. The beta and 95% confidence intervals in the forest plot ( a ) is shown for the SNP × physical activity interaction term, i.e., it indicates the decrease in LDL cholesterol levels in the active group as compared to the inactive group per each T allele of rs190748049. The −log 10 ( P value) in the association plot ( b ) is also for the SNP × physical activity interaction term. The P values are two-sided and were obtained using a meta-analysis of linear regression model results. The figure was generated using LocusZoom ( http://locuszoom.org ) Full size image No interaction between known main effect lipid loci and PA Of the previously known 260 main effect loci for HDL-C, 202 for LDL-C, and 185 for TG [3] , [4] , [5] , [6] , [7] , [8] , [9] , [10] , [11] , [12] , none reached the Bonferroni-corrected threshold (two-sided P INT = 1.0 × 10 −4 ) for SNP × PA interaction alone (Supplementary Data 4 - 6 ). We also found no significant interaction between a combined score of all published European-ancestry loci for HDL-C, LDL-C, or TG with PA (Supplementary Datas 7 – 9 ) using our European-ancestry summary results (two-sided P HDL-C = 0.14, P LDL-C = 0.77, and P TG = 0.86, respectively), suggesting that the beneficial effect of PA on lipid levels may be independent of genetic risk [15] . Potential functional roles of the loci interacting with PA While the mechanisms underlying the beneficial effect of PA on circulating lipid levels are not fully understood, it is thought that the changes in plasma lipid levels are primarily due to an improvement in the ability of skeletal muscle to utilize lipids for energy due to enhanced enzymatic activities in the muscle [16] , [17] . Of the four loci we found to interact with PA, three, in CLASP1 , near LHX1 , and in SNTA1 , harbor genes that may play a role in muscle function [18] , [19] and lipid metabolism [20] , [21] . The lead variant rs2862183 (minor allele frequency (MAF) 22%) in the CLASP1 locus which interacts with PA on HDL-C levels is an intronic SNP in CLASP1 that encodes a microtubule-associated protein (Fig. 2 ). The rs2862183 SNP is associated with CLASP1 expression in esophagus muscularis ( P = 3 × 10 −5 ) and is in strong linkage disequilibrium ( r 2 > 0.79) with rs13403769 variant that shows the strongest association with CLASP1 expression in the region ( P = 7 × 10 −7 ). Another potent causal candidate gene in this locus is the nearby GLI2 gene which has been found to play a role in skeletal myogenesis [18] and the conversion of glucose to lipids in mouse adipose tissue [20] by inhibiting hedgehog signaling. The rs295849 (MAF 38%) variant near LHX1 interacts with PA on HDL-C levels. However, the more likely causal candidate gene in this locus is acetyl-CoA carboxylase ( ACACA ), which plays a crucial role in fatty acid metabolism [21] (Fig. 3 ). Rare acetyl-CoA carboxylase deficiency has been linked to hypotonic myopathy, severe brain damage, and poor growth [22] . The lead variant in the SNTA1 locus (rs141588480) interacts with PA on HDL-C and is an insertion only found in individuals of African (MAF 6%) or Hispanic (MAF 1%) ancestry. The rs141588480 insertion is in the SNTA1 gene that encodes the syntrophin alpha 1 protein, located at the neuromuscular junction and altering intracellular calcium ion levels in muscle tissue (Fig. 4 ). Snta1 -null mice exhibit differences in muscle regeneration after a cardiotoxin injection [19] . Two weeks following the injection into mouse tibialis anterior, the muscle showed hypertrophy, decreased contractile force, and neuromuscular junction dysfunction. Furthermore, exercise endurance of the mice was impaired in the early phase of muscle regeneration [19] . In humans, SNTA1 mutations have been linked to the long-QT syndrome [23] . The fourth locus interacting with PA is CNTNAP2 , with the lead variant (rs190748049) intronic and no other genes nearby (Fig. 5 ). The rs190748049 variant is most common in African-ancestry (MAF 8%), less frequent in European-ancestry (MAF 2%), and absent in Asian- and Hispanic-ancestry populations. The protein coded by the CNTNAP2 gene, contactin-associated protein like-2, is a member of the neurexin protein family. The protein is located at the juxtaparanodes of myelinated axons where it may have an important role in the differentiation of the axon into specific functional subdomains. Mice with a Cntnap2 knockout are used as an animal model of autism and show altered phasic inhibition and a decreased number of interneurons [24] . Human CNTNAP2 variants have been associated with risk of autism and related behavioral disorders [25] . Joint test of SNP main effect and SNP × PA interaction We found 101 additional loci that reached genome-wide significance in the 2df joint test of SNP main effect and SNP × PA interaction on HDL-C, LDL-C, or TG. However, none of these loci showed evidence of SNP × PA interaction ( P INT > 0.001) (Supplementary Data 10 ). All 101 main effect-driven loci have been identified in previous GWAS of lipid levels [3] , [4] , [5] , [6] , [7] , [8] , [9] , [10] , [11] , [12] . In this genome-wide study of up to 250,564 adults from diverse ancestries, we found evidence of interaction with PA for four loci, in/near CLASP1 , LHX1 , SNTA1 , and CNTNAP2 . Higher levels of PA enhanced the HDL cholesterol-increasing effects of CLASP1 , LHX1 , and SNTA1 loci and attenuated the LDL cholesterol-increasing effect of the CNTNAP2 locus. None of these four loci have been identified in previous main effect GWAS for lipid levels [3] , [4] , [5] , [6] , [7] , [8] , [9] , [10] , [11] , [12] . The loci in/near CLASP1 , LHX1 , and SNTA1 harbor genes linked to muscle function [18] , [19] and lipid metabolism [20] , [21] . More specifically, the GLI2 gene within the CLASP1 locus has been found to play a role in myogenesis [18] as well as in the conversion of glucose to lipids in adipose tissue [20] ; the ACACA gene within the LHX1 locus plays a crucial role in fatty acid metabolism [21] and has been connected to hypotonic myopathy [22] ; and the SNTA1 gene is linked to muscle regeneration [19] . These functions may relate to differences in the ability of skeletal muscle to use lipids as an energy source, which may modify the beneficial impact of PA on blood lipid levels [16] , [17] . The inclusion of diverse ancestries in the present meta-analyses allowed us to identify two loci that would have been missed in meta-analyses of European-ancestry individuals alone. In particular, the lead variant (rs141588480) in the SNTA1 locus is only polymorphic in African and Hispanic ancestries, and the lead variant (rs190748049) in the CNTNAP2 locus is four times more frequent in African-ancestry than in European-ancestry. Our findings highlight the importance of multi-ancestry investigations of gene-lifestyle interactions to identify novel loci. We did not find additional novel loci when jointly testing for SNP main effect and interaction with PA. While 101 loci reached genome-wide significance in the joint test on HDL-C, LDL-C, or TG, all of these loci have been identified in previous GWAS of lipid levels [3] , [4] , [5] , [6] , [7] , [8] , [9] , [10] , [11] , [12] , and none of them showed evidence of SNP × PA interaction. The 2df joint test bolsters the power to detect novel loci when both main and an interaction effect are present [14] . The lack of novel loci identified by the 2df test suggests that the loci showing the strongest SNP × PA interaction on lipid levels are not the same loci that show a strong main effect on lipid levels. In summary, we identified four loci containing SNPs that enhance the beneficial effect of PA on lipid levels. The identification of the SNTA1 and CNTNAP2 loci interacting with PA was made possible by the inclusion of diverse ancestries in the analyses. The gene regions that harbor loci interacting with PA involve pathways targeting muscle function and lipid metabolism. Our findings elucidate the role and underlying mechanisms of PA interactions in the genetic regulation of blood lipid levels. Study design The present study collected summary data from 86 participating cohorts and no individual-level data were exchanged. For each of the participating cohorts, the appropriate ethics review board approved the data collection and all participants provided informed consent. We included men and women 18–80 years of age and of European, African, Asian, Hispanic, or Brazilian ancestry. The meta-analyses were performed in two stages [13] . Stage 1 meta-analyses included 42 studies with a total of 120,979 individuals of European ( n = 84,902), African ( n = 20,487), Asian ( n = 6403), Hispanic ( n = 4749), or Brazilian ancestry ( n = 4438) (Supplementary Table 1 ; Supplementary Data 2 ; Supplementary Note 1 ). 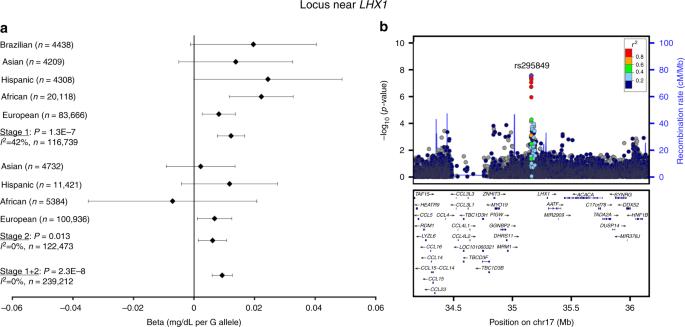Fig. 3 Interaction of rs295849 nearLHX1with physical activity on HDL cholesterol levels. The beta and 95% confidence intervals in the forest plot (a) is shown for the rs295849 × physical activity interaction term, i.e., it indicates the increase in logarithmically transformed HDL cholesterol levels in the active group as compared to the inactive group per each G allele of rs295849. The −log10(Pvalue) in the association plot (b) is also shown for the rs295849 × physical activity interaction term. ThePvalues are two-sided and were obtained by a meta-analysis of linear regression model results. The figure was generated using LocusZoom (http://locuszoom.org) Stage 2 meta-analyses included 44 studies with a total of 131,012 individuals of European ( n = 107,617), African ( n = 5384), Asian ( n = 6590), or Hispanic ( n = 11,421) ancestry (Supplementary Table 3 ; Supplementary Data 3 ; Supplementary Note 2 ). Studies participating in Stage 1 meta-analyses carried out genome-wide analyses, whereas studies participating in Stage 2 only performed analyses for 17,711 variants that reached P < 10 −6 in the Stage 1 meta-analyses and were observed in at least two different Stage 1 studies with a pooled sample size > 4000. The Stage 1 and Stage 2 meta-analyses were performed in all ancestries combined and in each ancestry separately. Outcome traits: LDL-C, HDL-C, and TG The levels of LDL-C were either directly assayed or derived using the Friedewald equation (if TG ≤ 400 mg dl −1 and fasting ≥ 8 h). We adjusted LDL-C levels for lipid-lowering drug use if statin use was reported or if unspecified lipid-lowering drug use was listed after 1994, when statin use became common. For directly assayed LDL-C, we divided the LDL-C value by 0.7. If LDL-C was derived using the Friedewald equation, we first adjusted total cholesterol for statin use (total cholesterol divided by 0.8) before the usual calculation. If study samples were from individuals who were nonfasting, we did not include either TG or calculated LDL-C in the present analyses. The HDL-C and TG variables were natural log-transformed, while LDL-C was not transformed. PA variable The participating studies used a variety of ways to assess and quantify PA (Supplementary Data 1 ). To harmonize the PA variable across all participating studies, we coded a dichotomous variable, inactive vs. active, that could be applied in a relatively uniform way in all studies, and that would be congruent with previous findings on SNP × PA interactions [26] , [27] , [28] and the relationship between PA and disease outcomes [29] . Inactive individuals were defined as those with <225 MET-min per week of moderate-to-vigorous leisure-time or commuting PA ( n = 84,495; 34% of all participants) (Supplementary Data 1 ). We considered all other participants as physically active. In studies where MET-min per week measures of PA were not available, we defined inactive individuals as those engaging in ≤1 h/week of moderate-intensity leisure-time PA or commuting PA. In studies with PA measures that were not comparable to either MET-min or hours/week of PA, we defined the inactive group using a percentage cut-off, where individuals in the lowest 25% of PA levels were defined as inactive and all other individuals as active. Genotyping and imputation Genotyping was performed by each participating study using Illumina or Affymetrix arrays. Imputation was conducted on the cosmopolitan reference panel from the 1000 Genomes Project Phase I Integrated Release Version 3 Haplotypes (2010–2011 data freeze, 2012-03-14 haplotypes). Only autosomal variants were considered. Specific details of each participating study’s genotyping platform and imputation software are described in Supplementary Tables 2 and 4 . Quality control The participating studies excluded variants with MAF < 1%. We performed QC for all study-specific results using the EasyQC package in R [30] . For each study-specific results file, we filtered out genetic variants for which the product of minor allele count (MAC) in the inactive and active strata and imputation quality [min(MAC INACTIVE ,MAC ACTIVE ) × imputation quality] did not reach 20. This removed unstable study-specific results that reflected small sample size, low MAC, or low-imputation quality. In addition, we excluded all variants with imputation quality measure <0.5. To identify issues with relatedness, we examined QQ plots and genomic control inflation lambdas in each study-specific results file as well as in the meta-analysis results files. To identify issues with allele frequencies, we compared the allele frequencies in each study file against ancestry-specific allele frequencies in the 1000 Genomes reference panel. To identify issues with trait transformation, we plotted the median standard error against the maximal sample size in each study. The summary statistics for all beta-coefficients, standard errors, and P values were visually compared to observe discrepancies. Any issues that were found during the QC were resolved by contacting the analysts from the participating studies. Additional details about QC in the context of interactions, including examples, may be found elsewhere [13] . Analysis methods All participating studies used the following model to test for interaction: 
    E[ Y ] = β _0 + β _E ∗ PA + β _G ∗ G + β _INT∗ G ∗ PA + β_c∗C,
 where Y is the HDL-C, LDL-C, or TG value, PA is the PA variable with 0 or 1 coding for active or inactive group, and G is the dosage of the imputed genetic variant coded additively from 0 to 2. The C is the vector of covariates which included age, sex, study center (for multi-center studies), and genome-wide principal components. From this model, the studies provided the estimated genetic main effect ( β G ), estimated interaction effect ( β GE ), and a robust estimate of the covariance between β G and β GE . Using these estimates, we performed inverse variance-weighted meta-analyses for the SNP × PA interaction term alone, and 2df joint meta-analyses of the SNP effect and SNP × PA interaction combined by the method of Manning et al. [14] , using the METAL meta-analysis software. We applied genomic control correction twice in Stage 1, first for study-specific GWAS results and again for meta-analysis results, whereas genomic control correction was not applied to the Stage 2 results as interaction testing was only performed at select variants. We considered a variant that reached two-sided P < 5 × 10 −8 in the meta-analysis for the interaction term alone or in the joint test of SNP main effect and SNP × PA interaction, either in the ancestry-specific analyses or in all ancestries combined, as genome-wide significant. The loci were defined as independent if the distance between the lead variants was >1 Mb. Combined PA-interaction effect of all known lipid loci To identify all published SNPs associated with HDL-C, LDL-C, or TG, we extended the previous curated list of lipid loci by Davis et al. [4] by searching PubMed and Google Scholar databases and screening the GWAS Catalog. After LD pruning by r 2 < 0.1 in the 1000 Genomes European-ancestry reference panel, 260 independent loci remained associated with HDL cholesterol, 202 with LDL cholesterol, and 185 with TG (Supplementary Datas 7 – 9 ). 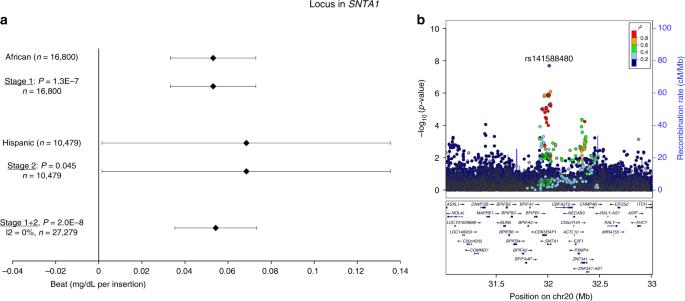Fig. 4 Interaction of rs141588480 inSNTA1with physical activity on HDL cholesterol levels. The beta and 95% confidence intervals in the forest plot (a) is shown for the rs141588480 × physical activity interaction term, i.e., it indicates the increase in logarithmically transformed HDL cholesterol levels in the active group as compared to the inactive group per each insertion of rs141588480. The –log10(pvalue) in the association plot (b) is also shown for the rs141588480 × physical activity interaction term. While the rs141588480 variant was identified in African-ancestry individuals in Stage 1, the variant did not pass QC filters in the Stage 2 African-ancestry cohorts, due to insufficient sample sizes of these cohorts. ThePvalues are two-sided and were obtained by a meta-analysis of linear regression model results. The figure was generated using LocusZoom (http://locuszoom.org) 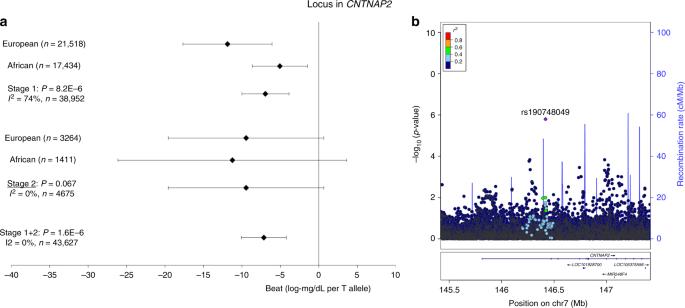Fig. 5 Interaction of rs190748049 variant inCNTNAP2with physical activity on LDL cholesterol levels. The rs190748049 variant was genome-wide significant in the joint test for SNP main effect and SNP × physical activity interaction and reachedP= 2 × 10−6for the SNP × physical activity interaction term alone. The beta and 95% confidence intervals in the forest plot (a) is shown for the SNP × physical activity interaction term, i.e., it indicates the decrease in LDL cholesterol levels in the active group as compared to the inactive group per each T allele of rs190748049. The −log10(Pvalue) in the association plot (b) is also for the SNP × physical activity interaction term. ThePvalues are two-sided and were obtained using a meta-analysis of linear regression model results. The figure was generated using LocusZoom (http://locuszoom.org) To approximate the combined PA interaction of all known European-ancestry loci associated with HDL-C, LDL-C, or TG, we calculated their combined interaction effect as the weighted sum of the individual SNP coefficients in our genome-wide summary results for European-ancestry. This approach has been described previously in detail by Dastani et al. [31] and incorporated in the package “gtx” in R . We did not weigh the loci by their main effect estimates from the discovery GWAS data. Examining the functional roles of loci interacting with PA We examined published associations of the identified lipid loci with other complex traits in genome-wide association studies by using the GWAS Catalog of the European Bioinformatics Institute and the National Human Genome Research Institute. We extracted all published genetic associations with r 2 > 0.5 and distance < 500 kb from the identified lipid-associated lead SNPs [32] . We also studied the cis -associations of the lead SNPs with all genes within ±1 Mb distance using the GTEx portal [33] . We excluded findings where our lead SNP was not in strong LD ( r 2 > 0.5) with the peak SNP associated with the same gene transcript.